DSIF and NELF interact with Integrator to specify the correct post-transcriptional fate of snRNA genes The elongation factors DSIF and NELF are responsible for promoter-proximal RNA polymerase II (Pol II) pausing. NELF is also involved in 3′ processing of replication-dependent histone genes, which produce non-polyadenylated mRNAs. Here we show that DSIF and NELF contribute to the synthesis of small nuclear RNAs (snRNAs) through their association with Integrator, the large multisubunit complex responsible for 3′ processing of pre-snRNAs. In HeLa cells, Pol II, Integrator, DSIF and NELF accumulate at the 3′ end of the U1 snRNA gene. Knockdown of NELF results in misprocessing of U1, U2, U4 and U5 snRNAs, while DSIF is required for proper transcription of these genes. Knocking down NELF also disrupts transcription termination and induces the production of polyadenylated U1 transcripts caused by an enhanced recruitment of cleavage stimulation factor. Our results indicate that NELF plays a key role in determining the post-transcriptional fate of Pol II-transcribed genes. In higher eukaryotes, transcripts produced by RNA polymerase II (Pol II) undergo one of three types of 3′ processing. While most protein-coding genes produce polyadenylated mRNAs, replication-dependent histone genes produce mRNAs lacking poly(A) tails and require a distinct set of cis elements and trans -acting factors for 3′ processing [1] , [2] . Pol II is also responsible for transcribing small, non-coding, non-polyadenylated small nuclear RNAs (snRNAs), which possess 3′ ends that are generated via a series of processing reactions starting with site-specific cleavage at an evolutionarily conserved 3′ box [3] . During the production of polyadenylated mRNAs, transcription and 3′ processing are tightly coupled; cleavage and polyadenylation factors are recruited during transcription, and transcript cleavage triggers transcription termination [2] , [4] , [5] . However, it is unclear whether this tight coupling holds true for the other types of 3′ processing. Moreover, little is known about the mechanisms by which the appropriate processing pathway is selected for a specific gene. Promoter-proximal pausing is a widespread checkpoint that occurs during the transcription cycle [6] , [7] , [8] . The elongation factors DSIF (comprising subunits Spt5 and Spt4) and NELF (comprising subunits NELF-A, -B, -C/D and -E) induce transcriptional pausing by interacting with early-elongation complexes. Positive transcription elongation factor b (P-TEFb) then phosphorylates the C -terminal domain (CTD) of Pol II at Ser2, thus reactivating the paused complex [9] , [10] , [11] , [12] , [13] . Furthermore, P-TEFb phosphorylates the C -terminal repetitive sequence (CTR) of DSIF, which is analogous to the Pol II CTD, and this modification converts DSIF from a transcriptional repressor to an activator [14] , [15] . A number of chromatin immunoprecipitation (ChIP) studies of Drosophila and mammals have supported the idea that NELF associates only with the 5′ end of protein-coding genes, while DSIF travels with Pol II throughout the elongation process [16] , [17] , [18] , [19] . However, recent studies have revealed that NELF also functions at the 3′ ends of certain genes to facilitate 3′ processing and/or transcription termination. For example, 3′ processing of histone genes requires binding of stem–loop-binding protein and U7 snRNP to evolutionarily conserved stem–loop and histone downstream elements, respectively, and is catalysed by cleavage and polyadenylation specificity factor (CPSF) [1] ; NELF interacts with the nuclear cap-binding complex and stem–loop-binding protein to facilitate histone-type 3′ processing [20] . Inhibition of these factors disrupts the canonical processing pathway and induces the production of aberrant polyadenylated histone mRNAs through the use of cryptic downstream poly(A) signals (PASs). Moreover, NELF is also involved in transcription termination of U2 snRNA [21] . Genes encoding snRNAs have TATA-less promoters that contain evolutionarily conserved distal and proximal sequence elements; these elements bind to Oct-1 and SNAPc/PTF, respectively, and direct transcription along with a set of general transcription factors and Pol II [22] . Primary snRNA transcripts are then cleaved, most likely co-transcriptionally, at a conserved 3′ box by Integrator, a 1.5-MDa complex that contains 12 subunits (Ints1–12), including two CPSF-like subunits [23] . Studies using kinase inhibitors and CTD mutants revealed that phosphorylation of the CTD at Ser2 and Ser7 is critical for this processing reaction [24] , [25] , [26] , [27] . Consistent with these findings, Integrator is able to bind tightly to the Pol II CTD phosphorylated at both Ser2 and Ser7 in vitro [28] . The present study was motivated by the identification of Integrator as a complex that interacts with both DSIF and NELF. Here we show that, along with Pol II and Integrator, DSIF and NELF accumulate at the 3′ end of the U1 snRNA gene and contribute to its synthesis in different ways. This study provides new insights into the mechanism by which the post-transcriptional fate of Pol II-transcribed genes is determined. DSIF and NELF interact with Integrator To understand the physiological roles of DSIF and NELF in more detail, proteins associated with Flag-tagged Spt5 (the large subunit of DSIF) and Flag-tagged NELF-E were affinity-purified from HeLa cell nuclear extracts and analysed using mass spectrometry ( Fig. 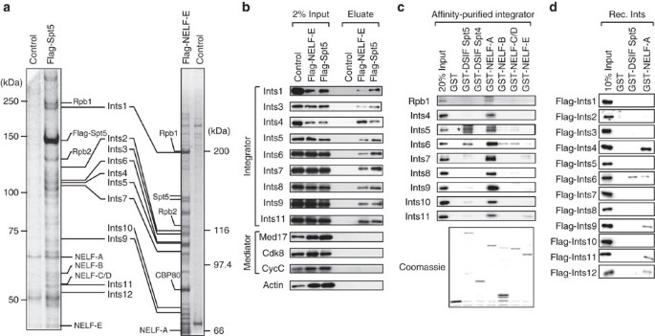Figure 1: DSIF and NELF interact with Integrator. (a) SDS–PAGE analyses of DSIF- and NELF-associated proteins affinity-purified from nuclear extracts of HeLa cells stably expressing Flag-Spt5 (left) or Flag-NELF-E (right). The extracts were also subjected to an LC-MS/MS analysis. See alsoSupplementary Table 1. (b) Immunoblot analyses of the samples described above using antibodies against specific subunits of Integrator and Mediator. Actin was detected as a loading control. (c,d) Equal amounts of GST or GST-tagged subunits of DSIF and NELF were immobilized to glutathione Sepharose beads and then incubated with Integrator affinity-purified from HeLa cells expressing Flag-Ints10 (c) or recombinant Integrator subunits expressed individually in insect cells (d). Rpb1 and the Integrator subunits were detected using immunoblotting. The asterisk denotes a nonspecific signal. See alsoSupplementary Fig. 1. Uncropped blots are shown inSupplementary Fig. 6. 1a and Supplementary Table 1 ). As expected, DSIF and NELF co-precipitated with each other and with Pol II. In addition, the cap-binding complex was co-purified with NELF, as reported previously [20] . Notably, 11 of the 12 subunits of Integrator, as well as C12orf11, which might be an additional subunit of Integrator [29] , [30] , were also co-purified with DSIF or NELF ( Fig. 1a and Supplementary Table 1 ). To exclude the possibility that the Integrator complex was co-purified due to interaction of DSIF and NELF with Pol II, the affinity-purified samples were analysed by immunoblotting with a panel of antibodies against subunits of Integrator and Mediator, the latter of which is another large protein complex that associates with Pol II. This experiment showed that Integrator subunits, but not Mediator subunits, co-precipitated with DSIF and NELF ( Fig. 1b ). Moreover, when Integrator was affinity-purified from HeLa cells expressing Flag-tagged Ints10, Spt5, NELF-E and the Pol II subunit Rpb1 were co-purified ( Supplementary Fig. 1a ), suggesting that Integrator interacts specifically with DSIF and NELF. Figure 1: DSIF and NELF interact with Integrator. ( a ) SDS–PAGE analyses of DSIF- and NELF-associated proteins affinity-purified from nuclear extracts of HeLa cells stably expressing Flag-Spt5 (left) or Flag-NELF-E (right). The extracts were also subjected to an LC-MS/MS analysis. See also Supplementary Table 1 . ( b ) Immunoblot analyses of the samples described above using antibodies against specific subunits of Integrator and Mediator. Actin was detected as a loading control. ( c , d ) Equal amounts of GST or GST-tagged subunits of DSIF and NELF were immobilized to glutathione Sepharose beads and then incubated with Integrator affinity-purified from HeLa cells expressing Flag-Ints10 ( c ) or recombinant Integrator subunits expressed individually in insect cells ( d ). Rpb1 and the Integrator subunits were detected using immunoblotting. The asterisk denotes a nonspecific signal. See also Supplementary Fig. 1 . Uncropped blots are shown in Supplementary Fig. 6 . Full size image To study these interactions under equilibrium conditions, HeLa cell nuclear extracts were subjected to sucrose gradient sedimentation analyses. The levels of DSIF, NELF, Integrator and Pol II components peaked in fraction number 11 (>1 MDa; Supplementary Fig. 1b ), suggesting the presence of a higher-order complex containing all of these factors. A large proportion of Ints3 was separated from the other Integrator subunits ( Supplementary Fig. 1b ). This additional peak may represent the recently identified SSOS complex that contains Ints3 and the human single-stranded DNA-binding protein homologues hSSB1 and hSSB2 (refs 31 , 32 , 33 , 34 ). DSIF and NELF interact with Integrator via Spt5 and NELF-A To determine whether DSIF and NELF interact directly with Integrator, pull-down assays were performed using affinity-purified Integrator and GST-tagged subunits of DSIF and NELF. GST-Spt5 and GST-NELF-A pulled down Integrator, although only Ints6 was co-precipitated efficiently by GST-Spt5 ( Fig. 1c ). Ints6 also interacted with GST-Spt5 in binding studies using insect cells expressing the 12 Integrator subunits individually ( Fig. 1d ), indicating a direct interaction between these proteins. In the same experiments, GST-NELF-A pulled down Ints4 most efficiently, whereas Ints6, Ints9, Ints11 and Ints12 were pulled down to a lesser extent ( Fig. 1d ). These data suggest that both DSIF and NELF interact directly with Integrator; the former probably occurs via binding of Spt5 to Ints6 and the latter likely occurs via binding of NELF-A to Ints4. The findings described above prompted us to investigate the role of the CTR, the CTD-like domain of Spt5, in Integrator binding. GST pull-down assays were performed using GST-Pol II CTD and GST-Spt5 CTR, with or without pre-phosphorylation by P-TEFb. Only the phosphorylated CTD was able to pull-down Integrator from HeLa nuclear extracts efficiently ( Supplementary Fig. 1c ), suggesting that the Spt5 CTR is not involved in Integrator binding. Inhibition of NELF induces misprocessing of snRNAs Next, we investigated the potential role of DSIF and NELF in 3′ processing of snRNAs in HeLa cells. Cleavage efficiency at the correct site was estimated using quantitative (q) RT–PCR using two sets of primers specific to total and cleaved snRNAs encoded by human RNU1 , RNU2 , RNU4 and RNU5 ( Fig. 2a ; RNU1 is shown as an example). Consistent with the results of previous studies [23] , [24] , [25] , [26] , inhibition of P-TEFb using Flavopiridol or short-hairpin RNA (shRNA)-mediated knockdown of Ints9, one of the CPSF-like subunits of Integrator, induced an accumulation of the uncleaved forms of U1, U2, U4 and U5, with only a minor effect on the total levels of these snRNAs, most of which are long-lived mature species ( Fig. 2b–d ). Knockdown of NELF using a NELF-E-specific shRNA also caused accumulation of the uncleaved forms of U1, U2, U4 and U5 in HeLa cells ( Fig. 2c,d ). To explore the possibility that the observed accumulation of the uncleaved forms of these snRNAs was because of an increase in their stability, the half-life of uncleaved U1 was determined by treating cells with the transcription inhibitor actinomycin D. The half-life of uncleaved U1 was not affected significantly by knockdown of NELF ( Supplementary Fig. 2a,b ), suggesting that NELF is involved in the cleavage of U1 pre-snRNA. By contrast, knockdown of Spt5 reduced the levels of the uncleaved forms of the U1, U2, U4 and U5 snRNAs ( Fig. 2c,d ), which may be attributable to the fact that DSIF contributes to transcription of the corresponding genes. 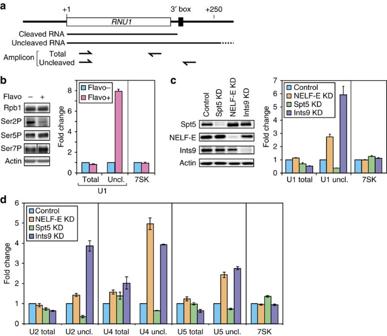Figure 2: Inhibiting P-TEFb, Integrator or NELF induces misprocessing of snRNAs. (a) Schematic illustration of the humanRNU1gene showing the positions of the primers used to amplify total and uncleaved U1 snRNA using qRT–PCR. (b) The left panel shows an immunoblot analysis of HeLa cells treated with DMSO (Flavo−) or 0.5 μM Flavopiridol (Flavo+) for 4 h. Antibodies specific for Rpb1 or Pol II phosphorylated at Ser2, Ser5 or Ser7 were used to confirm the inhibitory effect of Flavopiridol on P-TEFb. Actin was detected as a loading control. The right panel shows qRT–PCR analyses of total and uncleaved U1 snRNA in the same cells. (c) The left panel shows an immunoblot analysis of HeLa cells transfected with a control plasmid or a plasmid expressing a specific shRNAs to knockdown (KD) Spt5, NELF or Ints9. Cells were harvested for analysis 84 h after transfection. The right panel shows qRT–PCR analyses of total and uncleaved U1 snRNA in the same cells. (d) Quantitative RT–PCR analyses of the RNA samples shown incusing primers targeting theRNU2,RNU4andRNU5genes. (b–d) Expression of 7SK RNA was measured as an internal control in qRT–PCR experiments. The qRT–PCR data were normalized to those of the corresponding control cells and are represented as the mean±s.d. ofn=3 replicates. See alsoSupplementary Fig. 2. Uncropped blots are shown inSupplementary Fig. 7. Figure 2: Inhibiting P-TEFb, Integrator or NELF induces misprocessing of snRNAs. ( a ) Schematic illustration of the human RNU1 gene showing the positions of the primers used to amplify total and uncleaved U1 snRNA using qRT–PCR. ( b ) The left panel shows an immunoblot analysis of HeLa cells treated with DMSO (Flavo−) or 0.5 μM Flavopiridol (Flavo+) for 4 h. Antibodies specific for Rpb1 or Pol II phosphorylated at Ser2, Ser5 or Ser7 were used to confirm the inhibitory effect of Flavopiridol on P-TEFb. Actin was detected as a loading control. The right panel shows qRT–PCR analyses of total and uncleaved U1 snRNA in the same cells. ( c ) The left panel shows an immunoblot analysis of HeLa cells transfected with a control plasmid or a plasmid expressing a specific shRNAs to knockdown (KD) Spt5, NELF or Ints9. Cells were harvested for analysis 84 h after transfection. The right panel shows qRT–PCR analyses of total and uncleaved U1 snRNA in the same cells. ( d ) Quantitative RT–PCR analyses of the RNA samples shown in c using primers targeting the RNU2 , RNU4 and RNU5 genes. ( b – d ) Expression of 7SK RNA was measured as an internal control in qRT–PCR experiments. The qRT–PCR data were normalized to those of the corresponding control cells and are represented as the mean±s.d. of n =3 replicates. See also Supplementary Fig. 2 . Uncropped blots are shown in Supplementary Fig. 7 . Full size image To define the 5′ and 3′ ends of the read-through products in more detail and to provide a more quantitative perspective, absolute quantification of U1 transcripts in HeLa cells was performed using various primer sets and in vitro synthesized RNA as a standard. In control cells, the read-through products were expressed at 42±3 molecules per cell for +6/+196 RNA, 24±4 molecules per cell for +6/+418 RNA, 7.3±2.1 molecules per cell for +6/+658 RNA and 2.1±0.6 molecules per cell for +6/+911 RNA ( Supplementary Fig. 2c ). For reference, +21/+146 RNA, largely representing mature U1 snRNA, was present at 6.8±1.1 × 10 4 molecules per cell. On the other hand, transcripts upstream of the known transcription start site (TSS) of RNU1 were rare (1.4±0.3 molecules per cell for −90/+10 RNA), indicating that upstream transcription is negligible ( Supplementary Fig. 2c ). When NELF or Integrator was knocked down, the production of read-through products longer than 196 nt was induced 2.4- or 4.9-fold, respectively, whereas the production of transcripts longer than 911 nt was induced 5.8- to 6.7-fold, respectively ( Supplementary Fig. 2c ). These results indicate that longer read-through products are induced potently by knockdown of NELF or Integrator. Interplay of NELF, Integrator and DSIF on the U1 gene Next, we performed ChIP analysis of the RNU1 locus ( Fig. 3 ). Analysis of TBP showed that the resolution of our ChIP analysis was ~200 bp and that there was little overlap between ChIP signals from the 5′ and 3′ ends of the U1 gene ( Supplementary Fig. 3 ). In control HeLa cells, Pol II (Rpb4), DSIF (Spt5), NELF (NELF-A) and Integrator (Ints9) displayed a similar pattern of distribution on the U1 gene; a peak was identified at the 3′ end (b), and a very weak signal was detected at position +1250 relative to the TSS (e). The 5′ to 3′ signal ratios (a:b) of DSIF and NELF were reproducibly lower than that of Pol II, suggesting that these factors are recruited to the U1 gene at a later stage of transcription. 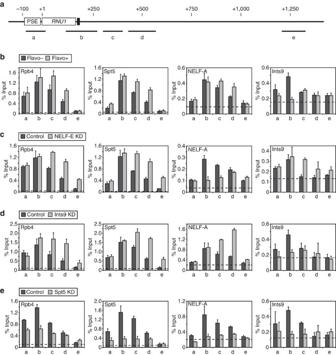Figure 3: Interplay of P-TEFb, NELF, Integrator and DSIF on theRNU1gene. (a) Schematic illustration of theRNU1locus showing the positions of the five amplicons used for ChIP analysis. The numbers are relative to the TSS. PSE, proximal sequence element. (b–e) ChIP analyses of the indicated proteins binding theRNU1locus. HeLa cells were treated with DMSO (Flavo−) or 0.5 μM Flavopiridol (Flavo+) for 4 h before harvesting (b). Alternatively, NELF-E (c), Ints9 (d) or Spt5 (e) was KD (as inFig. 2c) and soluble chromatin was prepared at 72 h post transfection. The data are represented as the mean±s.d. ofn=3 independent experiments. The dashed lines indicate background signals at an intergenic region of chromosome 2. See alsoSupplementary Fig. 3. Figure 3: Interplay of P-TEFb, NELF, Integrator and DSIF on the RNU1 gene. ( a ) Schematic illustration of the RNU1 locus showing the positions of the five amplicons used for ChIP analysis. The numbers are relative to the TSS. PSE, proximal sequence element. ( b – e ) ChIP analyses of the indicated proteins binding the RNU1 locus. HeLa cells were treated with DMSO (Flavo−) or 0.5 μM Flavopiridol (Flavo+) for 4 h before harvesting ( b ). Alternatively, NELF-E ( c ), Ints9 ( d ) or Spt5 ( e ) was KD (as in Fig. 2c ) and soluble chromatin was prepared at 72 h post transfection. The data are represented as the mean±s.d. of n =3 independent experiments. The dashed lines indicate background signals at an intergenic region of chromosome 2. See also Supplementary Fig. 3 . Full size image NELF is generally considered to act only at promoter-proximal regions. To determine whether recruitment of NELF to the 3′ region of the U1 gene is simply because of the small size of this gene or whether it reflects a functional difference between snRNA and protein-coding genes, we compared the NELF with Pol II signal ratios of the genes encoding U1 and beta-actin as a function of the distance from the TSS ( Supplementary Fig. 3 ). On the beta-actin gene, the normalized NELF signal around the TSS was higher than the corresponding signal at +300, which agrees with recent genome-wide NELF-binding studies showing that peak binding of this protein occurs close to the TSS [35] , [36] . Conversely, the normalized NELF signal around the TSS of the U1 gene was lower than the signals at positions +180 and +370 ( Supplementary Fig. 3 ). Thus, there is a subtle but definite difference in the distribution of NELF at these two gene loci. Knockdown of NELF in HeLa cells resulted in a marked relocalization of Pol II, DSIF and Integrator to the region downstream of the U1 gene ( Fig. 3c ). Together with the results of the qRT–PCR analysis ( Fig. 2c ), these findings suggest that knockdown of NELF causes profound defects in both 3′ processing and transcription termination of the U1 gene. Similar changes were also induced by knockdown of Ints9 ( Fig. 3d ) and, to a lesser extent, by Flavopiridol treatment ( Fig. 3b ). These data indicate that, as occurs for protein-coding genes, 3′ processing of the U1 gene is coupled to transcription termination. Furthermore, NELF, Integrator and P-TEFb appear to contribute to these processes. While inhibition of Pol II CTD Ser2 phosphorylation blocked the recruitment of Ints9 to the 3′ region of the U1 gene ( Fig. 3b ), knockdown of NELF had little effect on the recruitment of Ints9 to this region ( Fig. 3c ), and knockdown of Ints9 also had little effect on the recruitment of NELF to this region ( Fig. 3d ). When DSIF was knocked down, occupancy of the U1 gene by Pol II, NELF-A and Ints9 was reduced substantially ( Fig. 3e ). Under these conditions, knockdown of DSIF had little effect on the distribution of Pol II over the beta-actin gene (data not shown), suggesting that the knockdown did not have general, growth-related effects. These results are consistent with the notion that DSIF controls U1 gene transcription. It is unclear whether DSIF also contributes to the recruitment of NELF and Integrator, since knockdown of this protein results in a substantial reduction of Pol II occupancy. NELF inhibits aberrant polyadenylation of U1 transcripts The findings described above are reminiscent of what happens during 3′ processing of histone pre-mRNAs, another class of non-polyadenylated Pol II transcripts. Knockdown of NELF or a component of the histone 3′ processing machinery blocks histone pre-mRNA cleavage at the correct sites, resulting in an accumulation of aberrant polyadenylated histone mRNAs [20] , [37] , [38] . Therefore, RNA ligase-mediated rapid amplification of cDNA ends (RLM-RACE), which was modified to ensure that only transcripts with six or more adenosines at the 3′ ends were amplified ( Fig. 4a ), was used to determine whether aberrant polyadenylation of U1 transcripts also occurs as a result of knockdown of NELF. Quantitative TaqMan PCR analyses showed that knockdown of NELF or Integrator in HeLa cells induced the production of polyadenylated U1 transcripts but did not affect polyadenylation of GAPDH transcripts at the correct site ( Fig. 4b ). 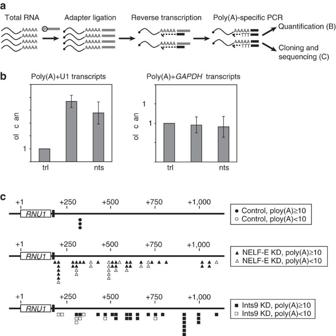Figure 4: Inhibition of NELF or Integrator leads to the accumulation of aberrant polyadenylated U1 transcripts. (a) Schematic representation of the RLM-RACE procedure. (b) TaqMan PCR analyses of poly(A)+ U1 transcripts and poly(A)+GAPDHtranscripts in control (Ctrl) HeLa cells and HeLa cells transfected with shRNAs to KD NELF-E or Ints9. The expression levels were normalized to the amount of 7SK RNA and to those of the control cells. Data are represented as the mean±s.e.m. ofn=5 independent experiments. *P<0.05 and **P<0.01 (two-tailed Student’st-test). (c) Cryptic polyadenylation sites of theRNU1gene. Untemplated poly(A) tails were detected in 3/48, 50/96 and 34/96 of the control, NELF-E knockdown and Ints9 knockdown clones, respectively. The polyadenylation sites of the positive clones were mapped on theRNU1locus. Clones containing short poly(A) tails (<10 nt) and those containing long poly(A) tails (⩾10 nt) are indicated by open and closed symbols, respectively. See alsoSupplementary Fig. 4. Figure 4: Inhibition of NELF or Integrator leads to the accumulation of aberrant polyadenylated U1 transcripts. ( a ) Schematic representation of the RLM-RACE procedure. ( b ) TaqMan PCR analyses of poly(A)+ U1 transcripts and poly(A)+ GAPDH transcripts in control (Ctrl) HeLa cells and HeLa cells transfected with shRNAs to KD NELF-E or Ints9. The expression levels were normalized to the amount of 7SK RNA and to those of the control cells. Data are represented as the mean±s.e.m. of n =5 independent experiments. * P <0.05 and ** P <0.01 (two-tailed Student’s t -test). ( c ) Cryptic polyadenylation sites of the RNU1 gene. Untemplated poly(A) tails were detected in 3/48, 50/96 and 34/96 of the control, NELF-E knockdown and Ints9 knockdown clones, respectively. The polyadenylation sites of the positive clones were mapped on the RNU1 locus. Clones containing short poly(A) tails (<10 nt) and those containing long poly(A) tails ( ⩾ 10 nt) are indicated by open and closed symbols, respectively. See also Supplementary Fig. 4 . Full size image Next, RLM-RACE products were cloned and sequenced to map the polyadenylation sites. Clones with fewer than six untemplated adenosine residues at their 3′ end were excluded from the analyses. A large number of polyadenylation sites were identified in the NELF knockdown and Integrator knockdown samples ( Fig. 4c and Supplementary Fig. 4 ). There was no detectable PAS (AAUAAA or its variants) around these sites. The absence of a PAS is not surprising because no PAS-like sequences are present in the 1-kb region downstream of the 3′ box of the U1 gene, where transcription termination mainly occurs. On the other hand, only a single polyadenylation site was identified from the control sample ( Fig. 4c and Supplementary Fig. 4 ). NELF prevents the recruitment of cleavage stimulation factor The findings described above raised a question as to whether aberrant polyadenylation is carried out by the canonical mRNA 3′-processing machinery. To address this question, CPSF-73 and the cleavage stimulation factor CstF-64 were knocked down by transfection of HeLa cells with recombinant lentiviruses expressing specific shRNAs ( Fig. 5a ). Knockdown of CPSF-73 resulted in a significant decrease in the amount of polyadenylated U1 transcripts, while knockdown of CstF-64 did not ( Fig. 5b ). Moreover, double knockdown studies showed that the accumulation of the polyadenylated U1 transcripts in NELF knockdown cells was reversed by concurrent knockdown of CPSF-73 or CstF-64 ( Fig. 5b ), suggesting that NELF prevents CPSF- and CstF-mediated cleavage and polyadenylation of U1 transcripts. 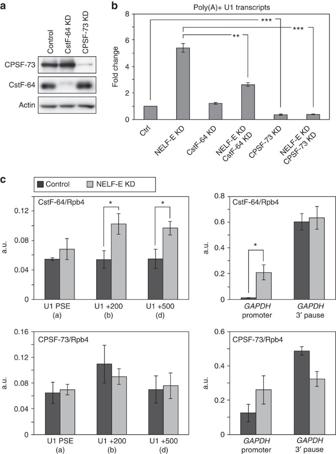Figure 5: NELF inhibits aberrant polyadenylation of U1 transcripts by preventing the recruitment of CstF-64. (a) Immunoblot analyses of HeLa cells transduced with recombinant lentiviruses expressing no shRNA (Control) or shRNAs designed to KD CstF-64 or CPSF-73. The cells were harvested at 7 days post infection. Actin was detected as a loading control. (b) TaqMan PCR analyses of poly(A)+ U1 transcripts and poly(A)+GAPDHtranscripts in control (Ctrl) HeLa cells and HeLa cells transfected with shRNAs to KD NELF-E, CstF-64 or CPSF-73. The expression levels were normalized to the amount of 7SK RNA and to those of the control cells. Data are represented as the mean±s.e.m. ofn=4 independent experiments. **P<0.01 and ***P<0.001 (two-tailed Student’st-test). (c) ChIP analyses of control HeLa cells and HeLa cells transfected with a shRNA to KD NELF. The ChIP assays were performed as described inFig. 3. After background subtraction, the ChIP signals of CstF-64 and CPSF-73 were normalized to those of Rpb4. The data are represented as the mean±s.e.m. ofn=5 (CstF-64/Rpb4) orn=3 (CPSF-73/Rpb4) independent experiments. *P<0.05 (two-tailed Student’st-test). See alsoSupplementary Fig. 5. Uncropped blots are shown inSupplementary Fig. 8. Figure 5: NELF inhibits aberrant polyadenylation of U1 transcripts by preventing the recruitment of CstF-64. ( a ) Immunoblot analyses of HeLa cells transduced with recombinant lentiviruses expressing no shRNA (Control) or shRNAs designed to KD CstF-64 or CPSF-73. The cells were harvested at 7 days post infection. Actin was detected as a loading control. ( b ) TaqMan PCR analyses of poly(A)+ U1 transcripts and poly(A)+ GAPDH transcripts in control (Ctrl) HeLa cells and HeLa cells transfected with shRNAs to KD NELF-E, CstF-64 or CPSF-73. The expression levels were normalized to the amount of 7SK RNA and to those of the control cells. Data are represented as the mean±s.e.m. of n =4 independent experiments. ** P <0.01 and *** P <0.001 (two-tailed Student’s t -test). ( c ) ChIP analyses of control HeLa cells and HeLa cells transfected with a shRNA to KD NELF. The ChIP assays were performed as described in Fig. 3 . After background subtraction, the ChIP signals of CstF-64 and CPSF-73 were normalized to those of Rpb4. The data are represented as the mean±s.e.m. of n =5 (CstF-64/Rpb4) or n =3 (CPSF-73/Rpb4) independent experiments. * P <0.05 (two-tailed Student’s t -test). See also Supplementary Fig. 5 . Uncropped blots are shown in Supplementary Fig. 8 . Full size image To test this proposal, the effect of knockdown of NELF on the recruitment of CPSF and CstF to the U1 gene was examined ( Fig. 5c and Supplementary Fig. 5 ). Knockdown of NELF increased the ratio of CstF-64 to Pol II at regions downstream of the U1 gene significantly (b and d), while the ratio of CPSF-73 to Pol II was only affected negligibly. These results suggest that NELF inhibits aberrant polyadenylation of U1 transcripts by preventing the recruitment of CstF to the U1 gene locus. Notably, knockdown of NELF also resulted in a significant increase in the relative ChIP signal of CstF-64 at the promoter region but not the 3′ region of the GAPDH gene ( Fig. 5c and Supplementary Fig. 5 ). Therefore, NELF may also prevent the recruitment of CstF to the promoter-proximal region of protein-coding genes. On the basis of the results of this study, we offer a model for transcription-coupled 3′ processing of snRNA genes ( Fig. 6 ). In this model, after the transcription initiation (step 1), DSIF (Spt4–Spt5) is recruited to Pol II to stimulate transcription elongation, while P-TEFb phosphorylates the Pol II CTD (step 2). Integrator is then recruited to the snRNA gene through its interactions with the phosphorylated-CTD and possibly DSIF. NELF is also recruited by DSIF and contributes to 3′ box-dependent 3′ processing by preventing the recruitment of CstF (step 3). Finally, Integrator performs 3′ processing and triggers transcription termination (step 4). 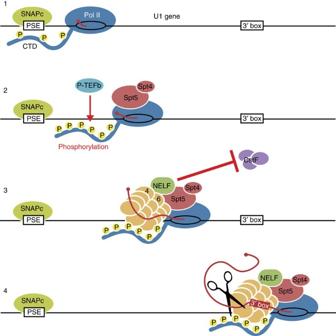Figure 6: Proposed model of the functions of DSIF, NELF and Integrator duringU1gene transcription and 3′ processing. After the transcription initiation (step 1), DSIF (Spt4–Spt5) is recruited to Pol II, while P-TEFb phosphorylates the Pol II CTD (step 2). Integrator is then recruited through its interactions with the phosphorylated-CTD and possibly DSIF. NELF is also recruited and contributes to 3′ box-dependent 3′ processing by preventing the recruitment of CstF (step 3). Finally, Integrator performs 3′ processing and triggers transcription termination (step 4). Figure 6: Proposed model of the functions of DSIF, NELF and Integrator during U1 gene transcription and 3′ processing. After the transcription initiation (step 1), DSIF (Spt4–Spt5) is recruited to Pol II, while P-TEFb phosphorylates the Pol II CTD (step 2). Integrator is then recruited through its interactions with the phosphorylated-CTD and possibly DSIF. NELF is also recruited and contributes to 3′ box-dependent 3′ processing by preventing the recruitment of CstF (step 3). Finally, Integrator performs 3′ processing and triggers transcription termination (step 4). Full size image Processing and termination at the 3′ end are tightly coupled during transcription of protein-coding genes, and, according to the widely accepted torpedo model, termination is induced by the 5′ to 3′ exoribonuclease Xrn2, which attacks the newly formed 5′ end of cleaved pre-mRNAs [4] , [5] . Since inhibition of NELF, Integrator and P-TEFb all resulted in defective 3′ processing and termination of the U1 gene ( Figs 2 and 3 ), it is likely that these processes occur in a coordinated manner by a mechanism similar to that of protein-coding genes. This view is consistent with a recent study that suggested the coupling of transcription termination and 3′ processing of U1 snRNA [39] . A few pieces of evidence suggest that DSIF is involved in U1 gene transcription. Specifically, knockdown of DSIF reduced the levels of both nascent (unstable) and processed (stable) U1 snRNA transcripts ( Fig. 2 ) and reduced the Pol II density across the RNU1 locus ( Fig. 3e ). Since DSIF functions as a dual regulator of transcription elongation for protein-coding genes, it may play a similar role in regulating the U1 gene. It may seem strange that an elongation factor is critical for the synthesis of such a small RNA; however, recent studies have shown that the little elongation complex, which comprises ELL and a few other subunits, is also required for the initiation and elongation phases of snRNA gene transcription [40] , [41] . It is not immediately clear why elongation factors are required for transcription of short snRNA genes. One possible reason is that elongation factors may maintain an open chromatin structure of highly transcribed snRNA genes. The binding pattern of histone H3 over the RNU1 and RNU2 genes is opposite to that of Pol II (refs 21 , 39 and our unpublished data), suggesting transcription-dependent eviction of histones. DSIF may contribute to a high level of expression of snRNA genes by counteracting the formation of a repressive chromatin structure. Since Integrator is implicated not only in 3′ processing of snRNAs but also in transcription of their genes per se [23] , [26] , [42] , it is also possible that DSIF contributes to snRNA transcription by interacting and cooperating with Integrator. On the basis of the results of recent genome-wide studies, NELF is generally considered to bind only to promoter-proximal regions [35] . However, our previous study showed that NELF is accumulated at both the 5′ and 3′ ends of replication-dependent histone genes and facilitates histone-type 3′ processing [20] . Moreover, NELF is accumulated at regions downstream of the U1 and U2 genes (refs 21 , 39 and this study). These findings led us to hypothesize that, aside from its established role in promoter-proximal pausing, NELF may also play a distinct role in the regulation of snRNA and histone genes. Unlike most Pol II-transcribed genes, snRNA and histone genes produce non-polyadenylated transcripts that follow the ‘minor’ 3′ processing pathways, and knockdown of NELF results in the production of aberrant polyadenylated species (ref. 20 and this study). Therefore, we speculate that polyadenylation is the default 3′ processing pathway and that NELF plays a key regulatory role in the post-transcriptional fate of Pol II-transcribed genes. As to the mechanism of aberrant polyadenylation, cryptic PASs are almost always located downstream of replication-dependent histone genes and are utilized when NELF or the histone-specific processing pathway is blocked. Polyadenylated histone mRNAs are stable but are not fully functional because they are not properly regulated during the cell cycle [37] , [43] . The cryptic PASs of histone genes may serve to ensure transcription termination and to prevent read-through into downstream genes. By contrast, PAS-like sequences were not identified within the region comprising a few kilobases downstream of the snRNA genes examined here. Despite the absence of a consensus PAS, polyadenylation of U1 transcripts apparently occurs at random when NELF or Integrator is knocked down ( Fig. 4c and Supplementary Fig. 4 ). This aberrant processing is dependent on CstF and CPSF ( Fig. 5 ), but it remains unclear which enzyme is responsible for poly(A) addition. Analysis of the half-life of U1 read-through products suggested that polyadenylated U1 transcripts are not very stable ( Supplementary Fig. 2a,b ). In Saccharomyces cerevisiae , the TRAMP complex attaches short oligo(A) tails to cryptic unstable transcripts and targets them for degradation by the nuclear exosome [44] , while mammalian homologues of TRAMP complex components have not been well characterized. Since U1 transcripts with both long and short poly(A) tails were identified by sequencing of RLM-RACE products ( Fig. 4c and Supplementary Fig. 4 ), aberrant polyadenylation may involve both canonical nuclear poly(A) polymerase and the TRAMP complex. The findings presented here suggest that NELF inhibits aberrant polyadenylation of U1 transcripts by preventing the recruitment of CstF. Regarding the mechanism by which CstF is recruited under normal circumstances, a recent study showed that Ser-65-phosphorylated TFIIB binds to and recruits CstF-64 to some protein-coding genes [45] . Another report suggested that CstF-50 interacts with the Pol II CTD in a phosphorylation-independent manner [46] . The way in which NELF interferes with the recruitment of CstF-64 to the U1 gene is an interesting but as yet unanswered question. Notably, knockdown of a histone-specific 3′ processing factor results in an increased association of CstF-50 with histone gene loci [47] . Therefore, the recruitment of CstF may be a common critical step in the determination of the post-transcriptional fate. Here we showed that knockdown of NELF also results in an increased association of CstF-64 with the 5′ end but not the 3′ end of the GAPDH gene ( Fig. 5c and Supplementary Fig. 5b ). Hence, NELF appears to exclude CstF from the promoter-proximal region of protein-coding genes while bound to Pol II, implying that a similar mechanism operates in both snRNA and protein-coding genes. Although a more detailed study is necessary to confirm the hypothesis, NELF may function to prevent premature termination at cryptic PASs located close to the TSSs of protein-coding genes. In fact, recent studies point to a new role of U1 snRNP in the suppression of premature termination [48] , [49] . Base-pairing of U1 snRNP to pre-mRNAs protects them from premature polyadenylation and transcription termination at nearby cryptic PASs within introns. To provide an integrated view of the post-transcriptional role of NELF, future studies will be aimed at reinvestigating the role of NELF in controlling protein-coding genes at a post-transcriptional level. Cell culture HeLa cells stably expressing Flag-NELF-E or Flag-Spt5 were generated as described previously [14] , [50] . HeLa cells stably expressing Flag-Ints10 were established by transfecting the cells with a pcDNA3-based expression vector and selecting neomycin-resistant colonies for 2 weeks. Nuclear extracts were prepared from HeLa cells using Dignam’s method. Analyses of protein–protein interactions Anti-Flag affinity purification was performed as described previously [20] . Briefly, NE buffer (20 mM HEPES-NaOH (pH 7.9), 20% glycerol, 100 mM KCl, 0.2 mM EDTA and 0.1% NP-40) was used for the binding and washing steps. Bound proteins were eluted with the same buffer containing 0.1 mg ml −l Flag peptide, excised from Coomassie-stained SDS polyacrylamide gels and subjected to LC-MS/MS analysis. Sucrose density-gradient centrifugation was performed as described previously [51] . For GST pull-down assays, GST fusion proteins and recombinant P-TEFb were prepared as described previously [14] , [20] , [52] . Affinity-purified Integrator was prepared from HeLa cells expressing Flag-Ints10, as described above. Recombinant Integrator subunits with an N -terminal Flag tag were expressed in Sf9 cells using the baculovirus expression system. Integrator was incubated with equal amounts of GST or GST fusion proteins immobilized to glutathione Sepharose (GE Healthcare) for 2 h at 4 °C. After extensive washing, bound materials were eluted with Laemmli buffer and analysed by immunoblotting. In Supplementary Fig. 1c , equal amounts of GST, GST-Pol II CTD or GST-DSIF CTR were immobilized to glutathione Sepharose and then incubated with or without recombinant P-TEFb and ATP for 10 min at 30 °C. After removal of P-TEFb and ATP, the matrices were incubated with HeLa nuclear extract in the presence of phosphatase inhibitor cocktail (Sigma) for 2 h at 4 °C. After extensive washing, bound materials were eluted with Laemmli buffer and analysed by immunoblotting. Immunoblotting Immunoblotting was performed according to the standard procedures using the following primary antibodies: anti-Flag M2 (Sigma, 5 μg ml −l ), anti-Rpb1 8WG16 (Covance, 1:1,000), anti-Spt5 (in-house, rabbit polyclonal, 1:1,000), anti-NELF-E (in-house, mouse monoclonal, 1 μg ml −1 ), anti-Ints1 (A300–361A, Bethyl, 1 μg ml −1 ), anti-Ints3 (A300–427A, Bethyl, 1 μg ml −1 ), anti-Ints4 (A301-296A, Bethyl, 0.2 μg ml −1 ), anti-Ints5 (A301-268A, Bethyl, 0.2 μg ml −1 ), anti-Ints6 (A300-254A, Bethyl, 0.2 μg ml −1 ), anti-Ints7 (A300-271A, Bethyl, 0.2 μg ml −1 ), anti-Ints8 (A300-269A, Bethyl, 1 μg ml −1 ), anti-Ints9 (A300-412A, Bethyl, 0.5 μg ml −1 ), anti-Ints10 (15271-1-AP, ProteinTech, 0.4 μg ml −1 ), anti-Ints11 (A301-274A, Bethyl, 0.2 μg ml −1 ), anti-Med17 (ARP34192, Aviva, 0.5 μg ml −1 ), anti-Cdk8 (RB-018, NeoMarkers, 1 μg ml −1 ), anti-Cyclin C (RB-009, NeoMarkers, 2 μg ml −1 ), anti-Ser2P H5 (Covance, 1:1,000), anti-Ser5P H14 (Covance, 1:3,000), anti-Ser7P 4E12 (Millipore, 1:3,000), anti-actin (MAB1501, Millipore, 0.2 μg ml −1 ), anti-CstF-64 (sc16473, Santa Cruz, 1 μg ml −1 ), and anti-CPSF-73 (A301-091A, Bethyl, 0.2 μg ml −1 ). RNA preparation and qRT–PCR Total RNA was prepared using Sepasol I Super (Nacalai Tesque) and then treated with RQ1 RNase-free DNase (Promega). Subsequently, qRT–PCR analyses were performed using the QuantiTect SYBR Green RT–PCR Kit (Qiagen), an ABI 7300 real-time PCR system (Applied Biosystems), and the primers listed in Supplementary Table 2 . RLM-RACE The RLM-RACE procedure was modified to ensure that only transcripts with six or more adenosines at the 3′ end were amplified [53] . First, RNA ligase was used to ligate a 5′ phosphorylated RNA/DNA chimeric oligonucleotide to the 3′ ends of transcripts in the total RNA sample, prepared as described above. Reverse transcription was then performed with a complementary DNA oligonucleotide and Superscript III reverse transcriptase (Life Technologies). Next, first-round PCR was carried out using a U1-specific forward primer and the same reverse primer amended to contain three additional adenosine residues at the 3′ end. Nested PCR was then performed using another U1-specific primer and a reverse primer with six adenosine residues. For cleavage site mapping, second-round PCR products of 250–2,000 bp were recovered from agarose gels, digested with Bam HI and Hin dIII, and then cloned into pBluescript SK+. In total, 48 or 96 clones were sequenced, most of which harboured RNU1-1 , RNU1–2 or RNU1–3 . Sequence analyses indicated that some clones were derived from transcripts with 3′ A-rich sequences rather than from polyadenylated transcripts; these irrelevant clones were excluded from further analyses. To quantify polyadenylated species of potentially variable lengths, first-round PCR products were subjected to TaqMan real-time PCR analyses. Gene knockdown using shRNAs The shRNA sequences were cloned into a version of pBluescript containing the mouse U6 promoter, as described previously [14] . The following sequences were used as shRNA targets: Spt5, 5′-AAGAACUGGGCGAGUAUUACA-3′; NELF-E, 5′-AAGAUGGAGUCAGCAGAUCAG-3′; Ints9, 5′-AAGAUCGAGAUCAUGCCAGAG-3′; CstF-64, 5′-AAGACCAAGAGACAGCACUUA-3′; and CPSF-73, 5′-AAGAUUCUGUAACACUGUCCA-3′. To knock down Spt5, NELF-E and Ints9, HeLa cells were transfected with a control plasmid (U6 promoter alone) or the specific shRNA-containing plasmid using Lipofectamine 2000 (Life Technologies), and transfectants were harvested at 72 h (for RNA analysis) or 84 h (for ChIP) post transfection. To knockdown CstF-64 and CPSF-73, a cassette containing the mouse U6 promoter and the specific shRNA sequence was excised from pBluescript and subcloned into pLenti6 (Life Technologies), as described previously [51] . Recombinant lentiviruses were produced according to the manufacturer’s recommendations and were used to infect HeLa cells. Infectants were selected in growth medium containing 4 μg ml −1 blasticidin and were harvested at 7 days post infection. ChIP assays ChIP assays were performed as described previously [14] . Briefly, HeLa cells were crosslinked with 1% formaldehyde for 10 min. Nuclei were isolated and resuspended in lysis buffer (10 mM Tris–HCl, pH 8.0, 100 mM NaCl, 1 mM EDTA, 0.5 mM EGTA, 0.1% SDS, protease inhibitor cocktail (Nacalai Tesque)). Chromatins were sheared by sonication using a Misonix S-4000 sonicator (Misonix). Soluble chromatins were incubated overnight at 4 °C with antibodies described below. Immunocomplexes were captured by protein G Sepharose FF (GE Healthcare) or Dynabeads Protein G (Dynal). Beads were sequentially washed three times with RIPA buffer (10 mM Tris–HCl, pH 8.0, 150 mM NaCl, 1 mM EDTA, 0.5 mM EGTA, 0.1% SDS, 1% Triton X-100, 0.1% sodium deoxycholate), three times with high-salt ChIP wash buffer (10 mM Tris–HCl, pH 8.0, 500 mM NaCl, 1 mM EDTA, 0.5 mM EGTA, 0.1% SDS, 1% Triton X-100, 0.1% sodium deoxycholate), twice with LiCl ChIP wash buffer (10 mM Tris–HCl, pH 8.0, 250 mM LiCl, 1 mM EDTA, 1 mM EGTA, 1% NP-40, 1% sodium deoxycholate), twice with TE (10 mM Tris–HCl, pH 8.0, 1 mM EDTA). Immunoprecipitates were eluted with elution buffer (100 mM NaHCO 3 , 1% SDS, 10 mM DTT) and incubated overnight at 65 °C. Genomic DNA fragments in inputs and eluates were purified and analysed using qPCR. The antibodies used for the assays were as follows: 2.5 μl of anti-Rpb4 sera (a gift from Koji Hisatake, University of Tsukuba; rabbit polyclonal), 2.5 μl of anti-Spt5 sera (in-house, rabbit polyclonal), 2.5 μl of anti-NELF-A sera (in-house, rabbit polyclonal), 1 μg of anti-Ints9 (A300–412A, Bethyl), 1 μg of anti-CstF-64 (A301-092A, Bethyl) and 1 μg of anti-CPSF-73 (A301-091A, Bethyl). The primer sequences are listed in Supplementary Table 2 . How to cite this article: Yamamoto, J. et al . DSIF and NELF interact with Integrator to specify the correct post-transcriptional fate of snRNA genes. Nat. Commun. 5:4263 doi: 10.1038/ncomms5263 (2014).